Enhanced reading by training with imposed time constraint in typical and dyslexic adults Poor reading skills of developmental dyslexics persist into adulthood with standard remediation protocols having little effect. Nevertheless, reading improves if readers are induced to read faster. Here we show that this improvement can be enhanced by training. Training follows a multi-session procedure adapted to silent sentence reading, with individually set, increasingly more demanding, time constraints (letter-by-letter masking). In both typical and dyslexic adult readers, reading times are shortened and comprehension improves. After training, the dyslexic readers’ performance is similar to that of typical readers; moreover, their connected text reading times and comprehension scores significantly improve in standard reading tests and are retained at 6 months post training. Identical training without time constraints proves ineffective. Our results suggest that fluent reading depends in part on rapid information processing, which then might affect perception, cognitive processing and possibly eye movements. These processes remain malleable in adulthood, even in individuals with developmental dyslexia. Dyslexic readers, including adults with university-level education, are characterized by effortful reading, which is slower and often less accurate compared to their normally reading peers [1] , [2] , [3] . The persistence of reading deficits that continues into adulthood, despite accumulating experience, has been partly attributed to a reduction in brain plasticity beyond childhood. In line with this view, it has been suggested that remedial interventions would prove less effective in adults [1] . Nevertheless, there is increasing evidence for effective skill learning and skill memory consolidation processes in adults [4] , [5] , [6] , [7] , [8] , [9] . It has been proposed that adults are not impaired in skill acquisition or retention per-se (including language-related skills [8] ), but are rather more selective in consolidating the memory for skills compared with children or young animals [8] , [9] , [10] , [11] , [12] . The intervention protocol that we present in the current study is based on two conceptions. First, that fluency constitutes a critical parameter of skilled reading [13] and time constrained reading (that is, being forced to read at a rate faster than one’s habitual reading rate) can significantly improve, albeit only for the duration of the test, reading accuracy and comprehension (the ‘acceleration phenomenon’) [14] , [15] . Accelerated reading may reduce distractibility, circumvent working memory limitations, increase readers’ reliance on stimulus-driven word decoding [16] , [17] , enhance synchronization of brain systems [15] and may reduce reliance on frontal language areas [1] , [18] . Second, training protocols, with increasingly more demanding time constraints on task performance, enhance the acquisition of a number of perceptual discrimination skills in adults [4] , [5] , [19] , [20] , [21] , [22] and can improve basic processing routines [4] , [19] , [20] , [23] . School children, trained with speed reading, have improved reading fluency with no reduction of comprehension [24] . Here we describe a computerized reading acceleration training protocol that introduced time constraints, improved the reading comprehension and reading fluency skills of both adult dyslexic readers and adult typical readers. Gains were retained 6 months post training. Importantly, the reading skills of the dyslexic group showed larger gains from the training protocol. In addition, results for testing routine reading performance (T1 test) indicate that there is a discrepancy between reading skills ability and performance for both groups. Furthermore, it is possible that the acceleration training helped to close this gap by better synchronizing between the brain systems that are activated in reading [15] . However, this point needs to be clarified by a study which also uses brain imaging parameters. Improved and retention of reading performance The acceleration training ( r-acc ) enhanced reading performance in both standard printed reading tests and in the computerized training protocol in two groups of readers, adult dyslexic and adult normal readers. On standard reading tests of fluency and comprehension as well as in a standard word-list reading test, readers who received r-acc training showed significant gains. Moreover, most of these gains were well retained in both reading level groups at 6 months post training (Table 3; Fig. 1 , T3). 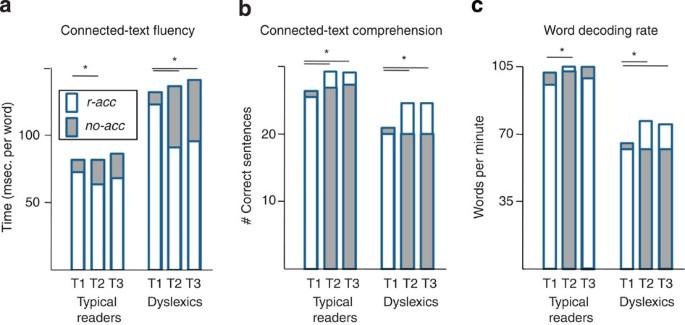Figure 1: Standard reading test performance of typical and dyslexic readers. Data are shown for three performance measures: (a) reading fluency for connected text; (b) number of correct responses to the comprehension questions (out of a total 30 questions); and (c) number of words decoded within a minute (word list). Note that followingr-acctraining (T2), both reading level groups, performed significantly better than the corresponding reading level-matched individuals who underwentno-acc-readtraining. Moreover, the dyslexic readers who hadr-acctraining performed at a level comparable to that of the typical readers who had nor-acctraining in terms of reading speed and comprehension of connected text. For each parameter alone,RM_analysis of variance with three test times(initial, final session and retention test at 6 months), as a within-Subject factor, andtwo Group(typical, dyslexic) andtwo Training(r-acc,no-acc-read), as between-Subject, factors *P<0.05 performed. Figure 1: Standard reading test performance of typical and dyslexic readers. Data are shown for three performance measures: ( a ) reading fluency for connected text; ( b ) number of correct responses to the comprehension questions (out of a total 30 questions); and ( c ) number of words decoded within a minute (word list). Note that following r-acc training (T2), both reading level groups, performed significantly better than the corresponding reading level-matched individuals who underwent no-acc-read training. Moreover, the dyslexic readers who had r-acc training performed at a level comparable to that of the typical readers who had no r-acc training in terms of reading speed and comprehension of connected text. For each parameter alone, RM_analysis of variance with three test times (initial, final session and retention test at 6 months), as a within-Subject factor, and two Group (typical, dyslexic) and two Training ( r-acc , no-acc-read ), as between-Subject, factors * P <0.05 performed. Full size image Although the dyslexic readers had lower scores than the typical readers, their r-acc training gains were significantly larger and better retained. ( Table 1 ; Fig. 2 , Figure 1 b ). Furthermore, the performance of the dyslexics undergoing r-acc training was close to that of typical readers receiving no reading acceleration ( no-acc-read ) training on both the immediate and the delayed post-training tests (T2, T3) ( Fig. 1b ). Table 1 Objective measures in standard reading tests. 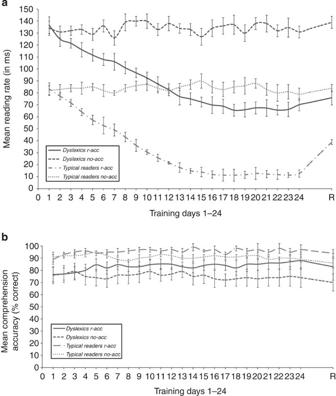Figure 2: The effects ofr-accpractice across 24 training sessions in typical and dyslexic readers. Group means for (a) reading rates and (b) comprehension accuracy. The per-letter reading rate was computed as the sentence reading time divided by the number of characters in the sentence. Comprehension accuracy is shown as a percentage of correct responses to the comprehension questions. Error bars represent standard deviation of the group means. Full size table Figure 2: The effects of r-acc practice across 24 training sessions in typical and dyslexic readers. Group means for ( a ) reading rates and ( b ) comprehension accuracy. The per-letter reading rate was computed as the sentence reading time divided by the number of characters in the sentence. Comprehension accuracy is shown as a percentage of correct responses to the comprehension questions. Error bars represent standard deviation of the group means. Full size image The effect of the r-acc training program on reading skills The parameters of the acceleration reading training programme also indicated robust gains in reading rate and comprehension ( Fig. 2a ). A repeated measures analysis of variance for per-letter reading time periods with Test time (initial, final), as within-Subject, and Group (typical, dyslexic) and Training ( r-acc , no-acc-read ), as between-Subject factors, showed significant improvement across training, but also a significant reading rate difference between groups, with the dyslexics slower than the typical readers ( Table 2 ). The type of training afforded was critical, as the gains in reading rate were exclusively expressed in participants training with time-constrained reading ( r-acc ) ( Table 2 ) ( Fig. 2a ). Overall, r-acc training was equally effective in the two reading level groups, but there were no significant gains in the no-acc-read training protocol ( Fig. 2a ). Table 2 Training and long-retention interval effects. Full size table During training, the comprehension scores in reading-masked sentences also improved significantly in all participants receiving r-acc training (76±6% to 87±7%, 89±4% to 97±5%, average±s.d., percent correct responses to comprehension questions within the initial and final sessions, dyslexic and typical readers, respectively), ( Table 2 ) ( Fig. 2b ). No such gains were found in either reading level group after no-acc-read training (76±7% to 75±8%, 91±4% to 89±3%, percent correct responses in initial and final sessions, dyslexic and typical readers, respectively), so that the gains accrued only in r-acc training (Table 2). The typical readers had significantly higher comprehension scores both before and after training ( Table 2 ; Fig. 2b ). However, the dyslexics gained more from r-acc training, compared with the typical readers. The training test parameters indicated that before training, the dyslexic readers assigned to r-acc training were significantly slower ( t (1,79)=5.97, P <0.001) and scored lower on the comprehension questions ( t (1,79)=4.21, P <0.001) compared with typical readers, with the slower reading rates negatively correlated with comprehension ( R =−0.598, P <0.001). However, in the final training sessions, dyslexic participants who had r-acc training had similar scores to the typical readers who had no-acc-read training, both in their per-letter reading rates and in the accuracy of responses to comprehension questions ( Fig. 2 ). Moreover, the gains were retained over a 6-month interval with the dyslexics showing somewhat better retention in terms of comprehension ( Table 2 b; Fig. 2 ). The imposition of time constraints on text reading during training was a crucial factor in improving reading skill in both reading-level groups. There are grounds to consider the possibility that the beneficial effects of training with time constrained masking relate to modifications of cognitive, motor, perceptual or word decoding routines specific to the skill of reading [25] , [26] , [27] . Poor reading is characterized by atypical ocular motor routines in reading [28] , such as more regressions and longer fixations, [29] , [30] and these routines may also be modified by training [29] , [30] , [31] , [32] , [33] . In adults, time-constrained training protocols have proved to be highly effective in inducing long-lasting gains in visual processing speed while improving discrimination [4] , [5] , [19] , [21] . Ineffective reading routines are implicated in explaining the discrepancy between accelerated and standard reading performance in dyslexic readers [15] . However, as our consistently negative results in the no-acc-read condition suggest, training in reading from a computer screen without imposed time constraints may engage the previously well-established reading routines (motor, perceptual or both), irrespective of reading level, in adults, rather than induce the establishment of new sub-routines. Nevertheless, training under task conditions that are far removed from the standard real-life reading experience may lead to expertise, which cannot be applied to standard reading performance [4] , [22] , [33] , [34] , [35] , [36] . Thus, the significant transfer of the r-acc -related gains to everyday text-reading performance indicates that the training experience engaged a level of processing that is of relevance to normal, unmasked and connected-text reading. In addition, the improvement of single word decoding as a result of the r-acc training among the two reading level groups may indicate a better access to and retrieval of word patterns from the mental lexicon and thus, may enhance connected-text reading rate and comprehension. Our findings also indicated that long-lasting retention of faster reading rate and higher comprehension was found within the two groups after r-acc training. The fact that the retention of the training effect was higher among the dyslexic readers, could instead of can be due to their lower initial reading skills, allowing them to gain much more in reading rate and comprehension. The current results indicate that the experience of reading with demanding, but manageable, time constraints may facilitate the establishment of additional improved text-processing sub-routines, even in highly experienced adults. Furthermore, our results indicate a behaviourally relevant potential for improving reading skills in adult dyslexics. Nevertheless, as the gap between the dyslexics’ performance vis-à-vis trained typical readers was clearly maintained after training, the current results suggest that r-acc , although highly effective, may not reset the life-long reading disability, but rather that a less-than-optimal reading routine was made more effective, for the dyslexics. This study focused adult, compensated dyslexics, and whether the training would bring about similar results for children must still be verified. Subjects A total of 110 university students, 55 recognized as dyslexic by the University of Haifa Clinic (Israeli Ministry of Education criteria, 2004), participated in the study. All dyslexic participants achieved mean reading scores of −1 s.d. and less in MATAL (2007) [39] standardized reading achievement test in Hebrew. The participants of both reading level groups (typical, dyslexic) were matched for age (22–29 years), gender (1:2, males/females), non-verbal IQ and level of education (2–4 years at the University) and had no indication of an attention deficit disorder (DSM 1994) [37] . Reading and reading-related standard tests performed before inclusion in the study showed that the dyslexics were significantly underperforming in all reading-related tests as well as in working memory capacity for words ( Table 3 ). Table 3 Reading and general ability measures at enrolment. Full size table Training protocol Forty participants of each reading level group were assigned to training in sentence reading with increasingly demanding time constraints (reading acceleration, r-acc ); 15 participants in each reading level group were assigned an identical amount of reading practice, with identical sentences, but with no time constraints (self-paced reading, no-acc-read ). All participants received 24 practice sessions (15–20 min each), three sessions per week with 1–3 days between-session intervals. In each session, 50 sentences (9–12 words, 45–70 letters, per sentence) were read, silently. The words were of medium-to-low frequency, ( http://atar.mscc.huji.ac.il/ ∼ frost/files/Word_frequency.xls ) in the un-pointed Hebrew script format. Each sentence was presented once throughout training. Participants were instructed to press a key as soon as they finished reading each sentence. A multiple-choice comprehension question followed. In order to overcome possible word length effects, time constraints (masking, r-acc ) were imposed using letter-by-letter erasure, advancing in the reading direction. Initial per-letter erasure rates were determined individually, from per-letter reading times in a 12 sentences pre-test (self-paced silent reading). Thereafter, erasure rate was increased or decreased by 2 ms per-character according to a stair-case procedure based on the number of consecutive comprehension questions correctly answered. Pre, post and long-post standard reading tests were obtained. Word decoding accuracy (Shatil, 1995) [38] , reading time for connected text and reading comprehension (MATAL, 2007) [39] were measured for all participants. How to cite this article : Breznitz, Z. et al. Enhanced reading by training with imposed time constraint in typical and dyslexic adults. Nat. Commun . 4:1486 doi: 10.1038/ncomms2488 (2013).